Enantioselective three-component aminomethylation of α-diazo ketones with alcohols and 1,3,5-triazines Enantioselective α -aminomethylation of carbonyl compounds constitutes a powerful protocol for introducing aminomethyl groups to simple organic molecules. However, current strategies rely on nucleophile-based enantioselective activation with inherently activated substrates only, and enantioselective protocol based on the activation of in situ-generated unstable formaldimines remains elusive, probably owing to their unstable nature and the lack of steric environment for efficient stereocontrols. Here, based on a rhodium/chiral phosphoric acid cooperative catalysis, we achieved an enantioselective three-component reaction of α -diazo ketones with alcohols and 1,3,5-triazines. A dual hydrogen bonding between the chiral phosphoric acid catalyst and two distinct active intermediates was proposed to be crucial for the efficient electrophile-based enantiocontrol. A series of chiral β -amino- α -hydroxy ketones including those derived from simple aliphatic alcohols, allylic alcohol, propargyl alcohol, complicated natural alcohols and water could all be prepared in high efficiency and enantioselectivity. As an important branch of Mannich reaction, the α -aminomethylation of carbonyl compounds constitutes a powerful protocol for introducing aminomethyl groups to simple organic molecules [1] , [2] , [3] , [4] , [5] , [6] , [7] , [8] . The resulting β -amino carbonyl compounds are versatile synthetic building blocks for a wide variety of natural products and biologically active compounds [9] . Different types of formaldehyde-derived imines or iminium salts, which are generally unstable and have to be in situ generated from formaldehyde with aromatic amines [10] , [11] , α -aminomethyl ethers [12] , [13] , [14] , [15] , [16] , [17] , N , O -acetals [18] , [19] , [20] , or 1,3,5-triaryl-1,3,5-triazines [21] , [22] , [23] , [24] , have been successfully applied. Within this context, enantioselective version of this transformation has also been achieved by catalytic asymmetric activation of the nucleophilic carbonyl compounds with either amine catalysts [10] , [11] , [14] , [16] or chiral Lewis acid [23] , [24] . While this nucleophile-based activating strategy was feasible and showed good enantiocontrol, the nucleophiles were limited to inherently activated substrates such as unmodified ketones or 1,3-dicarbonyl compounds (Fig. 1a , Eq 1). On the other hand, while the activation of stable imines by chiral Brønsted acid catalysts has been extensively investigated in a variety of enantioselective Mannich reactions [25] , [26] , [27] , [28] , [29] , [30] , [31] , [32] , [33] , [34] , [35] , [36] , this electrophile-based activating protocol has not been applied to aminomethylation reactions with the in situ-generated formaldimines, probably owing to their generally unstable nature and the lack of steric environment on the carbon atom for efficient stereocontrols (Fig. 1a , Eq 2). Fig. 1: Reaction design for aminomethylation with formaldimines. a Previous aminomethylation work of nucleophile activation mode. b Design of CPA dual hydrogen bonding directed electrophile activation mode multicomponent aminomethylation. Full size image In recent years, metal carbene-involved multicomponent reactions (MCRs) based on electrophilic trapping of active onium ylides have emerged as a powerful strategy to enable previously inefficient or even impossible chemical transformations [37] , [38] , [39] , [40] , [41] , [42] , [43] , [44] . Among them, the Mannich-type trapping of oxonium ylides with aryl imines has offered a rapid way for the synthesis of β -amino alcohols [45] , [46] , [47] , [48] . By utilizing rhodium/chiral phosphoric acid (CPA) cooperative catalysis, efficient stereocontrol via a crucial dual hydrogen bonding activation [34] , [49] , [50] from CPA toward both the oxonium ylide and the imine substrate has been achieved [45] , [46] , [48] . Encouraged by these discoveries, we design a three-component reaction between α -diazo ketones, alcohols and 1,3,5-triaryl-1,3,5-triazines, anticipating that a similar dual hydrogen bonding activation would be operational (Fig. 1b ), thus allowing an efficient electrophile-based asymmetric activation of formaldimines and offering an enantioselective aminomethylation reaction to give chiral β -amino- α -hydroxy ketones, which are widely existed structural scaffolds in synthetic and medicinal chemistry [51] , [52] , [53] , [54] . The challenges for the design of this three-component reaction are three-fold: (1) the in situ-generated formaldimine from 1,3,5-triazine has a low concentration in the reaction system, thus the electrophilic trapping of the active oxonium ylide species would be much less efficient and the undesired O–H insertion product [55] might be predominant; (2) 1,3,5-triaryl-1,3,5-triazines may undergo [4 + 1] cycloaddition with diazo compounds under metal catalysis [56] , which would lead to low reactivity of the desired three-component reaction; (3) it is not trivial whether the proposed dual hydrogen bonding between CPA and the two reactive intermediates could be effectively formed, which is owing to the unstable nature, low concentration and the lack of substituents on the carbon atom of the in situ-generated formaldimines. Reaction optimization By choosing 1,3,5-triphenyl-1,3,5-triazine 3a as the formaldimine precursor, initial screening of different diazo compounds was conducted with benzylic alcohol 1a under Rh(II)/phosphoric acid co-catalyzed conditions (For the initial screening of different diazo compounds, see Supplementary Fig. 1 in the Supplementary Information). 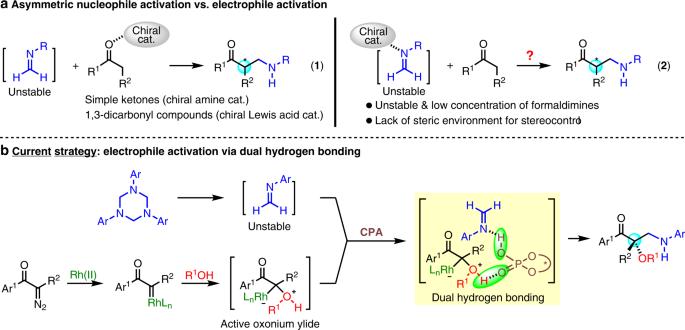Fig. 1: Reaction design for aminomethylation with formaldimines. aPrevious aminomethylation work of nucleophile activation mode.bDesign of CPA dual hydrogen bonding directed electrophile activation mode multicomponent aminomethylation. It was found that diazoacetophenone 2a reacted with 1a and 3a smoothly to afford three-component product 4a in 43% yield when Rh 2 (OAc) 4 and racemic phosphoric acid rac- 6a were employed as the co-catalysts (Table 1 , entry 1). In comparison, in the absence of CPA, the desired three-component product was not observed, instead, the [4 + 1] cyclization product 8 from 2a and 3a was obtained as the major product [56] . A series of CPAs were screened (entries 2–10), and the one possessing a bulky 3,3’-bis(2,4,6-triisopropylphenyl)-BINOL backbone [( R )- 6j ] showed most promising result, giving 4a in 61% yield with 74% ee (entry 10). When Rh 2 (OAc) 4 was replaced with Rh 2 (esp) 2 , both the yield and enantioselectivity were further improved (entry 11) (for a screening of different rhodium catalyst, see Supplementary Table 1 in the Supplementary Information). When 1-phenyl-diazoacetophenone 2b was used as the diazo source, the desired transformation occurred smoothly, affording 5a possessing a quaternary carbon center in 81% yield with 80% ee (entry 12). Introducing an ortho -trifluoromethyl substituent to the aryl ring of benzylic alcohol, as well as lowering the reaction temperature to −10 °C, allowed the corresponding three-component product 5b to be obtained in 81% yield with 94% ee (entries 13–14). Control experiments between 1b and 2b indicated that both rhodium and CPA catalysts were indispensable for this transformation (entries 15–16). Table 1 Condition optimization a . Full size table Substrate scope With the optimized reaction conditions in hand, the scope of this transformation was first investigated with different substituted benzylic alcohols (Fig. 2 ). Different ortho -substituents on the aryl ring of benzyl alcohols, including CF 3 , NO 2 , Cl, Br, I, MeO, Me, could be well tolerated, yielding the corresponding products in high yields with excellent ee ( 5b-5c , 5e-5i ). 1-Naphthylmethyl alcohol also worked well and showed excellent enantioselectivity ( 5j ). Non-substituted benzylic alcohol or the one bearing fluoro substituent at ortho -position gave the corresponding products with decreased ee ( 5a , 5d , 5k-5n ). These results indicated that the steric effects of the benzylic alcohol substrate, rather than its electronic properties, were more crucial for the enantiocontrol. Further increased bulkiness on the alcohol component completely inhibited the reactivity, indicating a strict balance between the steric effect and the reactivity of this transformation. Fig. 2: Substrate scope of benzylic alcohols. All reactions were run in 0.3 mmol scale of 1 , 1 : 2b : 3a = 1/1/0.33. All yields shown were based on isolated products. Ee values were determined by chiral HPLC analysis. Full size image The scope of 1,3,5-triaryl-1,3,5- triazines was then investigated by choosing 1-naphthylmethyl alcohol 1j as the alcohol (Fig. 3 ). In general, different substituents on the aryl ring of 1,3,5-triaryl-1,3,5-triazine, including Me, MeO, F, Cl, CF 3 , CO 2 Et at different positions, could all be well tolerated, yielding the corresponding products in moderate to good yields with excellent ee ( 5o - 5v ). Different substituted diazoacetophenones also worked well to give the desired products in good yields with excellent ee ( 5w and 5x ). The absolute configuration of 5o was unambiguously determined as S by single crystal X-ray analysis. Fig. 3: Substrates Scope of 1,3,5-Triaryl-1,3,5-triazines and diazo ketones. All reactions were run in 0.3 mmol scale of 1j , 1j : 2 : 3 = 1/1/0.33. All yields shown were based on isolated products. Ee values were determined by chiral HPLC analysis. Full size image In view of the great synthetic potential of the resulted chiral β -amino- α -hydroxy ketones, further efforts were made to expand the scope of alcohols (Fig. 4 ). Gratifyingly, by choosing diazoacetophenone 2a as the diazo source (For the screening of different diazo compounds, see Supplementary Fig. 2 in the Supplementary Information), aliphatic alcohols such as ethanol and 2-propanol reacted smoothly under standard conditions to give the corresponding products in moderate yields with high ee ( 4b and 4c ). Diarylmethanols also worked well to give the desired products with excellent ee ( 4d and 4e ) and the absolute configuration of the products derived from 2a was confirmed to be S by single crystal X-ray analysis of 4e . Allyl alcohol and propargyl alcohol were good substrates, affording the corresponding products in moderate to good yields with slightly decreased ee ( 4f and 4g ). The introduced allyl and propargyl groups offered a convenient way for further synthetic elaborations of the resulted β -amino ketones. Fig. 4: Substrates scope of different alcohols. Unless otherwise noted, the reactions were run in 0.3 mmol scale of 2a , 1 : 2a : 3a = 1/1/0.33. All yields shown were based on isolated products. Ee values were determined by chiral HPLC analysis. Dr values was determined by 1 H NMR of the crude reaction mixture. a The reactions were run in 0.3 mmol scale of 2a , 1 : 2a : 3 = 3/1/0.33. Full size image This method also offers an efficient protocol for the late-stage functionalization of complicated natural alcohols to introduce chiral β -amino- α -hydroxy ketone side chains. For example, geraniol and (2 E , 6 E )-farnesol were converted to corresponding three-component products in good yields with high ee ( 4h and 4i ). 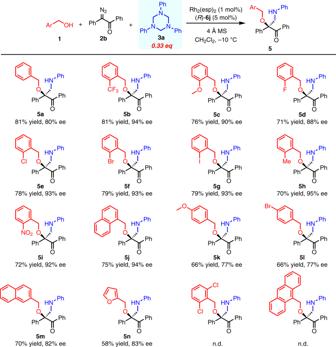Fig. 2: Substrate scope of benzylic alcohols. All reactions were run in 0.3 mmol scale of1,1:2b:3a= 1/1/0.33. All yields shown were based on isolated products. Ee values were determined by chiral HPLC analysis. (−)-Borneol and D -menthol also worked well to give desired product 4j and 4k in good yields with excellent dr. Cholesterol underwent this transformation to give the corresponding product 4l in 82% yield with 85:15 dr. To investigate the match/mismatch effect of this transformation, ( R )- 6j and ( S )- 6j were separately used as the catalyst for the three-component reactions of several chiral alcohols including (−)-borneol, D -menthol or L -menthol, reversed diastereoselectivities were generally observed (for detailed results, see Supplementary Table 2 in the Supplementary Information), indicating that the stereoselectivity of this transformation was mostly controlled by the chiral catalyst rather than the chiral substrate. The modification of commercial drugs and connection of two pharmaceutical fragments are useful for identifying potentially new drug molecules [57] , [58] , [59] , [60] . With the current strategy, an anti-HIV drug Darunavir [61] was successfully connected with cholesterol via a triazine formation/three-component reaction sequence, providing new compound 4m in high yield and dr (Fig. 5 ). 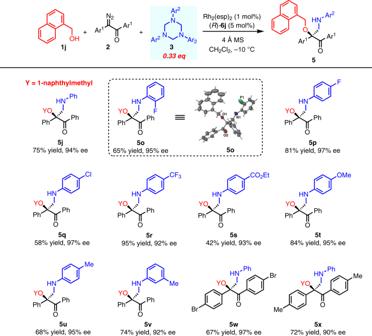Fig. 3: Substrates Scope of 1,3,5-Triaryl-1,3,5-triazines and diazo ketones. All reactions were run in 0.3 mmol scale of1j,1j:2:3= 1/1/0.33. All yields shown were based on isolated products. Ee values were determined by chiral HPLC analysis. Fig. 5: Drug linkage of Darunavir and cholesterol. Using Our protocol as a linkage tool reaction to connect Darunavir and cholesterol. Full size image More strikingly, water could be used as nucleophile to undergo current transformation to deliver the three-component product 4n in good yield and excellent ee (Fig. 6 ), thus offering a straightforward way to chiral β -amino- α -hydroxy ketones. Fig. 6: H 2 O derived three-component aminomethylation. Using water as nucleophile to directly afford O -unprotected β -amino- α -hydroxy ketone. Full size image Mechanistic studies To gain some insights into the pathway of this transformation, two control experiments were conducted. First, the O–H insertion product 7 derived from 1j and 2b was allowed to react with 3a under the optimal conditions, and the Mannich-type product 5j was not detected (Fig. 7a ). This result indicated that a stepwise O–H insertion/Mannich reaction pathway is unlikely involved in current transformation. On the other hand, the [4 + 1] cycloaddition product 8 derived from 2b and 3a , which has been observed as the major product when Rh(II) alone was used as the catalyst, failed to react with 1j under the optimal reaction conditions (Fig. 7b ), thus extruding the involvement of 8 as the intermediate for this transformation. Fig. 7: Mechanistic studies. a Control reaction to exclude the formation of product 5j from insertion product 7 . b Control reaction to exclude the formation of product 5j from cycloaddition product 8 . c , d Control reactions to verify the involvement of enol intermediate with diazo ketone 2e and 2e’ . Full size image In previously reported O–H insertion and rearrangement transformations between α -diazo ketones and alcohols, an enol intermediate has been proposed and characterized as the key intermediate [62] , [63] . Recent related DFT studies also supported the involvement of an enol intermediate in these processes [64] , [65] , [66] . To verify whether an enol intermediate was also involved for the current transformation, parallel experiments starting from 2-diazo-1-tetralone ( 2e ) or 1-diazo-2-tetralone ( 2e’ ) were conducted. For both reactions, the same three-component product 9 whose tertiary carbon was located at the 2-position were obtained as the major product (Fig. 7c, d ), indicating that an enol intermediate, rather than an oxonium ylide, might be involved for this transformation. In summary, a highly enantioselective three-component reaction of α -diazo ketones with 1,3,5-triazines and alcohols was developed under Rh(II)/chiral phosphoric acid cooperative catalysis. This reaction offers an efficient electrophile-based asymmetric activation mode of formaldimines for aminomethylation. A very broad scope of alcohols, including simple aliphatic alcohols, complicated natural alcohols and water, could all be applied, leading to a series of chiral β -amino- α -hydroxy ketones in good efficiency and high enantiocontrol. Efforts on understanding the stereocontrol of this transformation as well as applying this protocol to the trapping of other types of active intermediates are ongoing. General methods See Supplementary Methods for further details. Typical procedure for the aminomethylation reaction Under a nitrogen atmosphere, a suspension of Rh 2 (esp) 2 (1.0 mol%), chiral phosphoric acid ( R )- 6j (5 mol%), 4 Å molecular sieve (300 mg) was stirred in 2.0 mL of CH 2 Cl 2 at −10 °C and then the mixture of alcohol 1b (0.3 mmol), diazoacetophenones 2b (0.3 mmol) and 1,3,5-triaryl-1,3,5-triazinanes 3a (0.1 mmol) in 2 mL of CH 2 Cl 2 was introduced to the suspension over 2 h via a syringe pump. After completion of the addition, the reaction mixture was stirred for another 6 h until the diazo compound was completely consumed. The reaction mixture was then filtered through a short pad of Celite® and the filtrate was concentrated to give a residue which was subjected to HPLC for the ee values. Purification of the crude products by flash chromatography on silica gel (eluent: EtOAc/light petroleum ether = 1/80~1/40) afforded pure products ( S )- 5b . 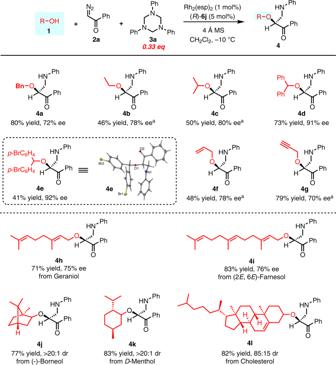Fig. 4: Substrates scope of different alcohols. Unless otherwise noted, the reactions were run in 0.3 mmol scale of2a,1:2a:3a= 1/1/0.33. All yields shown were based on isolated products. Ee values were determined by chiral HPLC analysis. Dr values was determined by1H NMR of the crude reaction mixture.aThe reactions were run in 0.3 mmol scale of2a,1:2a:3= 3/1/0.33. White solid, 81% yield, 94% ee, 1 H NMR (400 MHz, CDCl 3 ) δ 7.91 (s, 2 H), 7.69–6.99 (m, 14 H), 6.70–6.47 (m, 3 H), 4.88 (d, J = 10.1 Hz, 1 H), 4.38 (d, J = 10.1 Hz, 1 H), 4.08 (d, J = 12.5 Hz, 1 H), 3.87 (d, J = 12.1 Hz, 1 H), 3.81 (s, 1 H). 13 C NMR (101 MHz, CDCl 3 ) δ 199.80, 147.88, 138.96, 135.40, 134.59, 133.07, 131.82, 130.26, 130.11, 129.08, 128.92, 128.20, 128.13, 127.86, 125.83, 125.13, 117.36, 99.99, 87.31, 63.32, 47.80. 19 F NMR (376 MHz, CDCl 3 ) δ -59.68. 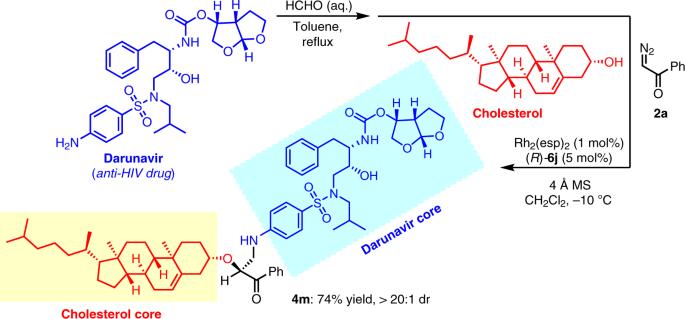Fig. 5: Drug linkage of Darunavir and cholesterol. Using Our protocol as a linkage tool reaction to connect Darunavir and cholesterol. HRMS: Calcd. 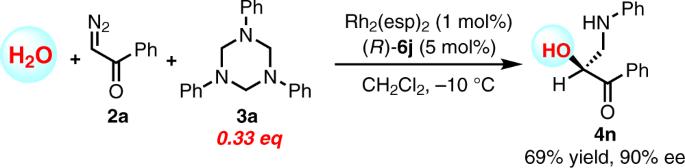Fig. 6: H2O derived three-component aminomethylation. Using water as nucleophile to directly affordO-unprotectedβ-amino-α-hydroxy ketone. 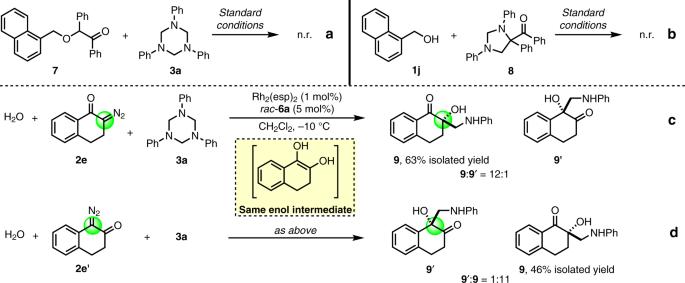Fig. 7: Mechanistic studies. aControl reaction to exclude the formation of product5jfrom insertion product7.bControl reaction to exclude the formation of product5jfrom cycloaddition product8.c,dControl reactions to verify the involvement of enol intermediate with diazo ketone2eand2e’. for C 29 H 25 F 3 NO 2 (M + H) + : 476.1837, found: 476.1804, HPLC (Chiral IA, λ = 254 nm, hexane/2-propanol = 20/1, Flow rate = 1.0 mL/min), t major = 5.81 min, t minor = 6.68 min.